Evidence for an oxygen evolving iron–oxo–cerium intermediate in iron-catalysed water oxidation The non-haem iron complex α -[Fe II (CF 3 SO 3 ) 2 (mcp)] (mcp=( N , N′ -dimethyl- N , N ′-bis(2-pyridylmethyl)-1,2- cis -diaminocyclohexane) reacts with Ce IV to oxidize water to O 2 , representing an iron-based functional model for the oxygen evolving complex of photosystem II. Here we trap an intermediate, characterized by cryospray ionization high resolution mass spectrometry and resonance Raman spectroscopy, and formulated as [(mcp)Fe IV (O)( μ -O)Ce IV (NO 3 ) 3 ] + , the first example of a well-characterized inner-sphere complex to be formed in cerium(IV)-mediated water oxidation. The identification of this reactive Fe IV –O–Ce IV adduct may open new pathways to validate mechanistic notions of an analogous Mn V –O–Ca II unit in the oxygen evolving complex that is responsible for carrying out the key O–O bond forming step. High-valent iron-oxo species are implicated in important biological and synthetic oxidative transformations [1] , [2] , [3] . Some of these species have also shown a remarkable competence towards water oxidation to form dioxygen, a reaction that involves O-O bond formation [4] , [5] , [6] , [7] . The reaction is particularly appealing because it has been recognized as one of the bottleneck challenges for the success of artificial photosynthesis, and the identification of iron compounds as efficient catalysts opens novel directions in the quest for earth-abundant systems that could be used on a large scale [8] , [9] , [10] , [11] . In this context, the study of the water oxidation (WO) reaction with chemical oxidants catalysed by well-defined coordination complexes can clarify fundamental principles underlying the mechanisms of O-O bond formation and cleavage [12] , [13] , the latter being at the heart of chemical processes by which aerobic organisms respire [14] . Most remarkably, given the strong parallels between the oxidation chemistry of iron and manganese compounds [15] , it can be envisioned that fundamental chemical insights extracted from studies of O-O bond formation by iron coordination compounds can shed light on intermediates and mechanisms operating at the Oxygen Evolving Complex (OEC). We and others have recently shown that non-haem iron complexes containing tetradentate nitrogen-based ligands are competent catalysts for chemically driven WO [4] , [5] , [16] , [17] . In our systematic studies, we determined that the presence of two cis labile sites is required for WO activity and that electronic effects modulate the catalytic efficiency, providing basic principles for catalyst design [4] , [5] . 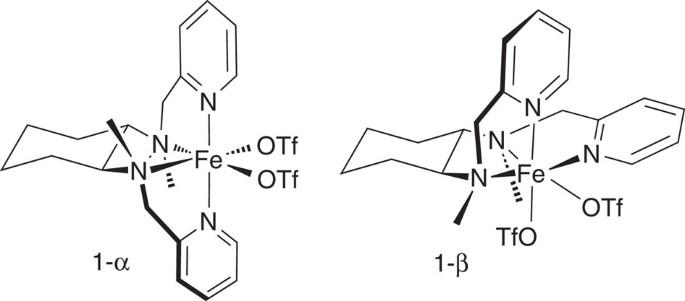Figure 1: Iron water oxidation catalysts. Schematic structure of the iron complexes used in this study. Herein, we present evidence for a catalytically relevant reaction intermediate that precedes the oxidation of the water molecule in the case of α -[Fe II (CF 3 SO 3 ) 2 (mcp)], 1- α ( Table 1 ), which we have identified as a particularly active catalyst. This transient species is characterized by high resolution mass spectrometry (CSI-HRMS) and resonance Raman spectroscopy (rR) as a heterodimetallic oxo-bridged iron-cerium complex formed by the reaction of the oxoiron(IV) complex α -[Fe IV (O)(H 2 O)(mcp)] 2+ and Ce IV . The Fe(O)( μ -O)Ce(OH 2 ) n core of this intermediate bears a strong structural resemblance to the Mn(O)( μ -O)Ca(OH 2 ) 2 unit found in the natural oxygen evolving centre. Most remarkably, the Fe(O)( μ -O)Ce(OH 2 ) n unit is catalytically competent in water oxidation. Table 1 Water oxidation catalytic activities for 1- α and 1- β . Full size table Catalytic activity of 1-α and 1-β in water oxidation [Fe II (CF 3 SO 3 ) 2 (mcp)] is known to form two topological isomers, 1- α and 1- β ( Fig. 1 ) [18] , [19] , [20] , [21] , which have previously been shown to behave differently as catalysts for C-H and C=C bond oxidations [19] , [21] . Given this sensitivity, the abilities of both complexes to act as water oxidation catalysts were explored. In a typical reaction, an aqueous solution of 1- α or 1- β (0.5 ml, 12.5 μM, final concentration) was added to an aqueous solution of CAN (9.5 ml, 125 mM, pH=0.8, final concentration and pH). Gases evolved from these reactions were monitored by manometry and quantified by gas chromatography with a thermal conductivity detector (GC-TCD). Under these conditions ( Table 1 ), 1- α was highly active and yielded 160±10 and 380±20 TON of O 2 , (mol of O 2 /mol of catalyst) when using 100 and 12.5 μM catalyst concentrations, respectively. In contrast, very small amounts of O 2 were detected when the same experiment was carried out with its topological isomer 1- β (4±1 and 5±2 TON, respectively). Therefore, despite the fact that the two complexes differed only in their ligand topology, their activities as water oxidation catalysts were found to be drastically different. Besides O 2 , only small amounts of CO 2 were present at the end of the reaction (<1 TON), indicating that no major ligand oxidation occurred during catalytic O 2 evolution. Figure 1: Iron water oxidation catalysts. Schematic structure of the iron complexes used in this study. Full size image Spectroscopic characterization Reactions were then analysed spectroscopically to gain insight into the origin of the marked differences in reactivity ( Fig. 2 ). The reaction of 1- α or 1- β with CAN (3 eq.) in H 2 O (final pH=1) resulted in the formation of α/β -[Fe IV (O)(H 2 O)(mcp)] 2+ , 2- α or 2- β , respectively. Both exhibited near-IR bands characteristic of Fe IV (O) complexes, namely λ max =769 nm ( ε =270 M −1 cm −1 ) for 2 -α and λ max =778 nm ( ε =280 M −1 cm −1 ) for 2 -β ( Fig. 2a,b and Supplementary Fig. 1-2 ). The use of 2.5 equivalents of Ce IV to fully transform 1 - α,β to 2- α,β may be an indication of the high redox potential necessary to oxidize Fe III -OH 2 to Fe IV (O) ( Fig. 3 ). Taking into consideration the Nernst equation, the redox potential for the Fe III -OH 2 /Fe IV (O) couple under the low pH reaction conditions is estimated at ~1.4 V versus NHE, which matches that obtained in recent DFT calculations [22] . 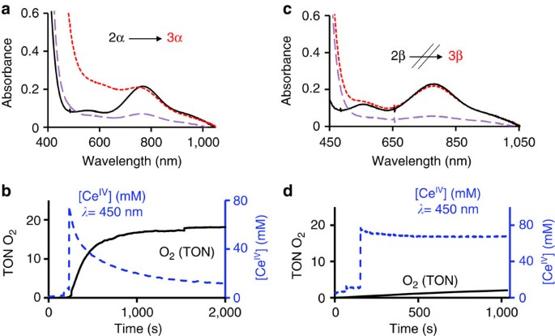Figure 2: Real-time manometry/UV–vis monitoring of oxygen evolution and cerium(IV) consumption. UV–vis spectra of (a)2-αand (c)2-β(solid black line) formed by the respective reactions of1-αand1-β(1 mM) in Milli-Q H2O at 25 °C with 3 equiv. of CAN, on addition of 75 equiv. of CAN (dotted red line) and after CAN consumption (dashed purple line). Time courses for the reaction of (b)1-αand (d)1-βwith 75 equiv. CAN monitoring, [CeIV] (right axis, dotted blue line), and O2evolution (left axis, solid black line). Kinetic traces for [CeIV] were monitored at 450 nm. Δ[O2] (TON) was monitored by a pressure transducer and quantified by GC-TCD. Figure 2: Real-time manometry/UV–vis monitoring of oxygen evolution and cerium(IV) consumption. UV–vis spectra of ( a ) 2 -α and ( c ) 2 -β (solid black line) formed by the respective reactions of 1- α and 1- β (1 mM) in Milli-Q H 2 O at 25 °C with 3 equiv. of CAN, on addition of 75 equiv. of CAN (dotted red line) and after CAN consumption (dashed purple line). Time courses for the reaction of ( b ) 1- α and ( d ) 1- β with 75 equiv. CAN monitoring, [Ce IV ] (right axis, dotted blue line), and O 2 evolution (left axis, solid black line). Kinetic traces for [Ce IV ] were monitored at 450 nm. Δ[O 2 ] (TON) was monitored by a pressure transducer and quantified by GC-TCD. 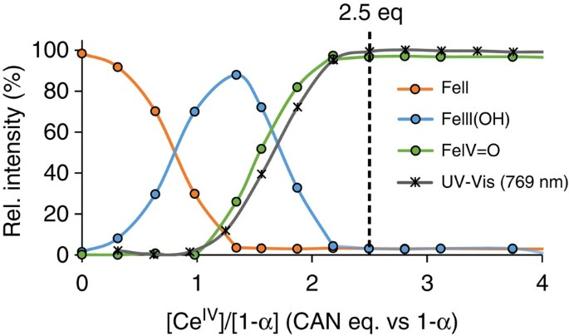Figure 3: FeII(OH2) to FeIV(O) titration with CeIVmonitored by UV–vis and HRMS. Distribution ofFeII,FeIIIandFeIVspecies according to relative ion peak intensities obtained by HRMS in the titration of2-αwith CeIV. The UV–vis titration (formation of FeIV=O monitored at 769 nm) was also superimposed in the plot (black crosses). Full size image Figure 3: Fe II (OH 2 ) to Fe IV (O) titration with Ce IV monitored by UV–vis and HRMS. Distribution of Fe II , Fe III and Fe IV species according to relative ion peak intensities obtained by HRMS in the titration of 2- α with Ce IV . The UV–vis titration (formation of Fe IV =O monitored at 769 nm) was also superimposed in the plot (black crosses). Full size image Formation of 2- α was further confirmed and monitored by CSI-HRMS ( Fig. 4a and Supplementary Figs 3–7 ) and 1 H-NMR spectroscopy (see Supplementary Figs 8 and 9 ). The excellent agreement between speciation observed by UV–vis and ESI-MS shows a clean transformation between 1-α and 2-α ( Fig. 3 ). Importantly, the CSI-HRMS spectra of 2- α showed an intense peak at m/z =545.110±0.003 that can be assigned to {[Fe IV (O)(mcp)](CF 3 SO 3 )} + on the basis of its m/z value and isotope distribution pattern. Consistently, the peak moved to 547.117±0.003 when 2- α was generated in H 2 18 O, due to the incorporation of 18 O into the oxo ligand. In addition, a second strong signal at m/z =413.162±0.003 was observed, which shifts to 417.172±0.003 when H 2 18 O was used. Therefore, the peak was assigned to the [Fe IV (O)(OH)(mcp)] + ion ( Supplementary Figs 3–7 ). These ions may correspond to the respective loss of H 2 O and CF 3 SO 3 H from the parent {[Fe IV (O)(OH 2 )(mcp)](CF 3 SO 3 )} + ion, thus identifying 2- α as [Fe IV (O)(OH 2 )(mcp)] 2+ . 2- α could be also prepared by reacting [Fe II (Cl) 2 (mcp)] with CAN (3 eq. ), providing further evidence for water and not a triflate ion as the sixth ligand. In addition, support for a terminal oxo ligand in 2- α was obtained by rR spectroscopy ( λ exc =413.1 nm, −8 °C, in 1:1 H 2 O:CH 3 CN), where a resonance enhanced feature was observed at 822 cm −1 . This feature downshifted by 40 cm −1 with the use of H 2 18 O ( Fig. 5a ), consistent with its assignment to the Fe=O stretch of 2- α [23] , [24] . 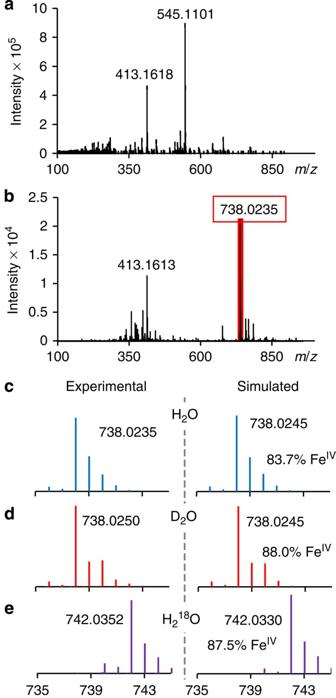Figure 4: Characterization of 3-αby high resolution mass spectrometry (a) CSI-HRMS spectrum of2-α, recorded immediately after the oxidation of1-α(1 mM) by CAN (3 mM). (b) CSI-HRMS spectrum obtained during the WO reaction, on the addition of 75 equiv. of CAN to2-α. (c–e) CSI-HRMS features associated with3-αobtained in H2O, D2O and H218O as solvent. Spectra were recorded by setting the nebulizer and dry gas temperature of the cryospray instrument to 25 °C. Figure 4: Characterization of 3- α by high resolution mass spectrometry ( a ) CSI-HRMS spectrum of 2- α , recorded immediately after the oxidation of 1- α (1 mM) by CAN (3 mM). ( b ) CSI-HRMS spectrum obtained during the WO reaction, on the addition of 75 equiv. of CAN to 2- α . ( c – e ) CSI-HRMS features associated with 3- α obtained in H 2 O, D 2 O and H 2 18 O as solvent. Spectra were recorded by setting the nebulizer and dry gas temperature of the cryospray instrument to 25 °C. 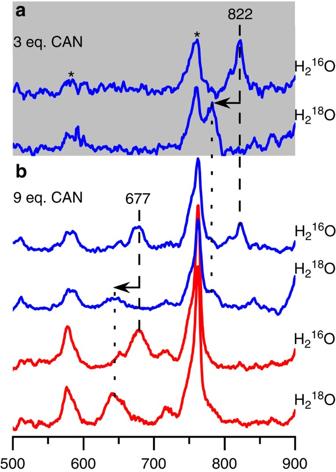Figure 5: Characterization of reaction intermediates by Resonance Raman. (a) Highlighted in grey, rR spectra of2-α(λex413.1 nm, 100 mW) prepared on addition of 3 equiv. CAN to a solution of1-α(5 mM) in 1:1 H2O:MeCN. (b) rR spectra of3-αprepared on addition of 9 equiv. CAN to a solution of1-αin 1:1 H2O:MeCN. Blue:λex=413.1 nm, 100 mW, [Fe]=5 mM. Red:λex=514.5 nm, 100 mW, [Fe]=8 mM. All spectra were collected from liquid solutions maintained at −8 °C. Asterisks denote features arising from CAN. The intensity of the MeCN solvent peak at 922 cm−1was used to normalize the intensities of the peaks among the various spectra. Full size image Figure 5: Characterization of reaction intermediates by Resonance Raman. ( a ) Highlighted in grey, rR spectra of 2- α ( λ ex 413.1 nm, 100 mW) prepared on addition of 3 equiv. CAN to a solution of 1- α (5 mM) in 1:1 H 2 O:MeCN. ( b ) rR spectra of 3- α prepared on addition of 9 equiv. CAN to a solution of 1- α in 1:1 H 2 O:MeCN. Blue: λ ex =413.1 nm, 100 mW, [Fe]=5 mM. Red: λ ex =514.5 nm, 100 mW, [Fe]=8 mM. All spectra were collected from liquid solutions maintained at −8 °C. Asterisks denote features arising from CAN. The intensity of the MeCN solvent peak at 922 cm −1 was used to normalize the intensities of the peaks among the various spectra. Full size image Decay of 2- α (τ 1/2 =20 min at 25 °C) did not result in O 2 evolution, showing that it cannot be the WO species. In fact, further reaction of 2- α with CAN was necessary to generate the WO species. To investigate the nature of the latter, the reaction of 2- α with an excess of CAN was monitored simultaneously by UV–vis spectroscopy, manometry and CSI-HRMS ( Fig. 6 , Supplementary Fig. 10 ). UV–vis spectroscopy and CSI-HRMS were used to monitor the time-dependent evolution of the oxoiron(IV) species, as well as the consumption of Ce IV , while O 2 evolution within the same time period was determined by manometry and GC-TCD. 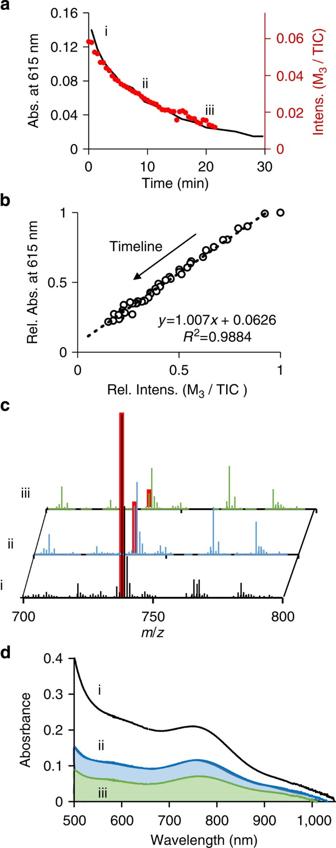Figure 6: Decay of 3-α monitored by UV–vis and HRMS. (a) Time course for the decay of the 615 nm chromophore (line, left axis) and theM3MS peak intensity (dots, right axis) during the reaction of1-α(1 mM) with CAN (75 mM) at 25 °C. (b) Correlation between the relative absorbance (Abst/Abs0) at 615 nm and ion count [(M3/TIC)t/(M3/TIC)0] ofM3. (t=time of measurement;. TIC=total ion count). (c,d) Mass and visible spectra observed at 10 s (i), 10 min (ii) and 20 min (iii) after the addition of CAN (75 equiv.) to2-α(1 mM in Milli-Q water, 25 °C). Figure 6: Decay of 3-α monitored by UV–vis and HRMS. ( a ) Time course for the decay of the 615 nm chromophore (line, left axis) and the M 3 MS peak intensity (dots, right axis) during the reaction of 1- α (1 mM) with CAN (75 mM) at 25 °C. ( b ) Correlation between the relative absorbance (Abs t /Abs 0 ) at 615 nm and ion count [( M 3 /TIC) t /( M 3 /TIC) 0 ] of M 3 . ( t =time of measurement;. TIC=total ion count). ( c , d ) Mass and visible spectra observed at 10 s (i), 10 min (ii) and 20 min (iii) after the addition of CAN (75 equiv.) to 2- α (1 mM in Milli-Q water, 25 °C). Full size image Reaction of CAN (75 equiv.) with 2- α resulted in O 2 evolution concomitant with Ce IV consumption. After all Ce IV was consumed, O 2 evolution stopped and 18.4 TON of O 2 ( Fig. 2c , Supplementary Fig. 10 ) were formed. Therefore, 98% of the added CAN was converted productively to O 2 , (maximum TON=18.75 based on the initial Ce IV with n(Ce IV )/n(O 2 )=4). At this point, 30% of the initial amount of 2- α remained in solution, as judged by its absorbance at λ =769 nm ( Supplementary Fig. 10d ). The CSI-HRMS spectrum of the solution showed intense peaks at m/z =414.1696 and 739.0270, values that are within experimental error of the exact masses for [Fe III (mcp)(OH) 2 ] + and [(mcp)Fe(O)(OH)Ce(NO 3 ) 3 ] + species, respectively; associated isotope distribution patterns are also consistent with these formulations. The addition of a second aliquot of CAN (75 equiv.) restarted O 2 evolution, producing an additional 11 TON of O 2 until Ce IV depletion ceased and complete disappearance of the 769 nm band ( 2- α ) was observed ( Supplementary Figs11,12 ). The reaction of 2- α with CAN (75 equiv.) elicited the immediate appearance of a broad absorption band in the 500-650 nm range and a hypsochromic shift of the near-IR feature of 2- α ( Fig. 2a , Supplementary Fig. 10b ). These changes were not observed on addition of triflic acid (TfOH), Ce III (NO 3 ) 3 or Sc(OTf) 3 to 2- α . Interestingly, the new chromophore gradually diminished in intensity concomitant with Ce IV consumption, and the near-IR band of 2- α re-emerged (albeit with a reduced intensity because of partial decomposition) ( Fig. 2a and Supplementary Fig. 10 ). These observations provide evidence for the accumulation of a novel reaction intermediate, 3- α . The formation of 3- α was further corroborated by a kinetic analysis of the reaction of 2- α with CAN at 25 °C and pH=1. The initial rates of Ce IV consumption and O 2 evolution by 1- α (0.1 mM) showed a saturation behaviour with respect to [Ce IV ]. In addition, the reaction rate exhibited a linear dependence on 2-α (0.01–1 mM), and in [Ce IV ] at [Ce IV ] in the 1.25–12.5 mM range, with a reaction order close to one for both reagents at large Ce/Fe ratios (under pseudo-first order conditions). At [Ce IV ]>12.5 mM, reaction rates exhibited saturation, becoming independent of [Ce IV ] (see Supplementary Figs 13–19 ). This kinetic behaviour indicates a pre-equilibrium binding of Ce IV to 2-α leading to the accumulation of an intermediate, namely 3-α , the evolution of which represents the rate determining step of the reaction. We assessed the viability of this notion by analysing the reaction between Ce IV and 2- α to form 3- α in 1:1 v-v CH 3 CN:H 2 O solution at −8 °C, a temperature at which O 2 evolution and Ce IV consumption basically ceased. We found that the formation of 3- α is very fast and reversible, with an equilibrium constant K eq of 120(±25) that could be estimated from the titration data (See Supplementary Figs 20–24 , Supplementary Tables 1 and 2 and Supplementary Methods ). Notably, analogous kinetic observations have been made in WO mediated by [Fe II (CF 3 SO 3 ) 2 ( Me,X Pytacn)] ( Me,X Pytacn=1-(2′-pyridylmethyl)-4,7-dimethyl-1,4,7-triazacyclononane, X=H, Cl, CO 2 Et, NO 2 ), suggesting the possibility of a common pathway for WO by these two non-haem iron WO catalysts [5] . Like 1- α , the topological isomer 1- β reacted with CAN (3 eq.) to form the S =1 β -[Fe IV (O)(OH 2 )(mcp)] 2+ ( 2- β , λ max =753 nm, ε =280 M −1 cm −1 ) as judged by UV–vis, CSI-HRMS and 1 H-NMR (See Supplementary Fig. 1 , right, Supplementary Figs 3, 8 and 9 ). However, in contrast to 2- α , the reaction of 2- β with CAN (75 equiv.) did not result in a significant decrease in the concentration of CAN nor was O 2 evolution observed ( Fig. 2d ). Moreover, the formation of a putative 3-β was not observed. Given the structural similarity between 2- α and 2- β , the failure of the latter to elicit water oxidation, together with the kinetic similarities between 2- α and the catalytically active [Fe II (CF 3 SO 3 ) 2 ( Me,X Pytacn)] complexes [5] , strongly suggests that the formation of 3- α is required for WO to proceed. Characterization of intermediate 3- α CSI-HRMS experiments shed some light on the nature of 3- α that was formed in the reaction of 2- α with Ce IV under catalytic conditions ([Fe]=1 mM; [CAN]=75 mM, Fig. 4 , Supplementary Figs 25 and 26 ). The addition of CAN caused the disappearance of the peak at m/z =545.110 corresponding to 2- α ( Fig. 4b ) and the appearance of a new peak at m/z 738.0235 and designated as M 3 , which was not observed when 1- β was treated with excess of CAN ( Supplementary Fig. 27 ). The composition of M 3 was deduced with the aid of isotopic labelling. When H 2 18 O was used as a solvent, M 3 upshifted by four units ( Fig. 4e ). As the oxygen atoms of the nitrates do not undergo fast exchange with H 2 18 O (see Supplementary Fig. 28 ), this upshift suggests that M 3 must contain two oxygen atoms capable of facile exchange with water. In contrast, experiments with D 2 O showed that M 3 does not have exchangeable protons ( Fig. 4d ). Furthermore, the isotopic distribution pattern of M 3 could only be correctly simulated by taking into account the natural abundance isotopes of one Fe and one Ce atom. Specifically, the 54 Fe isotope (5.8% relative to 56 Fe) is responsible for the M 3 –2 peak, while the 142 Ce isotope (11.1% relative to 140 Ce) contributes significantly to the M 3 +2 peak ( Supplementary Fig. 29 ). Taken together, these results allow M 3 to be formulated as {[Fe IV (O) 2 (mcp)Ce IV (NO 3 ) 3 ]} + (calc. m/z 738.0245, found m/z 738.0235) (For further details see Supplementary Methods ). This formulation requires the replacement of one hydrogen atom from the [Fe IV (O)(OH)(mcp)] + ion ( m/z 413.1616) by the [Ce IV (NO 3 ) 3 ] + moiety to give rise to M 3 . Collision induced dissociation (CID) MS/MS experiments at different collision energies (CE) were performed for M 3 ( m/z =738.0). At relative low energies (12 eV), the CID fragmentation of M 3 +H led to the loss of a neutral HNO 3 ( m/z =676.0). Only at CE higher than 24 eV did the parent peak at 738.0 disappear, but the m/z 676.0 ion (corresponding to neutral loss of HNO 3 from M 3 +H) persisted at even higher collision energies (up to 39 eV). These results indicate the robustness of the {Fe IV -O-Ce IV } moiety in the gas phase ( Supplementary Fig. 30 ). Decisively, Fig. 6 shows that the decay of M 3 (monitored by CSI-HRMS) parallels the decrease in the intensity of the 615 nm chromophore attributed to 3- α . Such a correlation indicates that M 3 in fact corresponds to 3- α . Taken together, the spectroscopic results and the kinetic model that arises from analysing Ce IV consumption and O 2 evolution establishes 3- α as the last detectable and catalytically competent intermediate in water oxidation. The molecular structure derived from the MS analysis indicates that 3- α corresponds to M 3 , but the ion may also contain additional water ligands bound at Ce(IV) in the solution state that would be readily lost in the gas phase. This proposal is supported by the fact that Ce(IV) forms kinetically labile and dynamic complexes with a coordination number of 8 to 9. Furthermore, recent Ce(IV) speciation and quantum dynamic studies have shown a fast ligand exchange at the coordination sphere of Ce(IV) [25] , [26] , [27] . More detailed insight into the nature of the iron-cerium adduct was provided by rR spectroscopy of liquid samples maintained at −8 °C in a 1:1 H 2 O:MeCN solvent mixture. UV–vis and mass spectrometry characterization of 2- α and 3- α in this solvent mixture indicates that their identities are the same as in pure water ( Supplementary Table 3 ). This temperature was employed to stabilize 3- α sufficiently so as to be characterized by rR. Furthermore, under these conditions, O 2 production also correlates with decay of 3- α ( Supplementary Fig. 31 ). As shown in Fig. 5 , the rR spectrum ( λ ex =413.1 nm, Fig. 5a ) of 2- α prepared with 3 equiv. of Ce IV exhibits a feature at 822 cm −1 that downshifts to 782 cm −1 on replacing H 2 16 O by H 2 18 O, consistent with its assignment to the ν Fe=O of 2- α . Near-UV excitation was required to observe this feature as 2- α has insignificant absorbance in the visible region, as found for other non-haem oxoiron(IV) complexes [23] , [24] . Interestingly, the rR spectra of 3- α obtained with the same excitation wavelength ( λ ex =413.1 nm, Fig. 5b ) also show the 822 cm −1 vibration and its downshift to 782 cm −1 upon H 2 18 O substitution. This feature may arise from either 2- α or 3- α or both species. To clarify, we compared the intensities of the 822 cm −1 peaks for the 2- α (3-CAN) and 3- α (9-CAN) samples relative to the adjacent 762-cm −1 nitrate feature as an internal standard, after taking into account that the 9-CAN sample has three times the amount of nitrate as the 3-CAN sample. Indeed, the two samples are found to have 822 cm −1 peaks of comparable intensity. Given an association constant of 120(±25) M −1 (in agreement with a K eq of 90(±10) M −1 under catalytic conditions, at 25 °C in H 2 O, obtained by the kinetic analysis of O 2 evolution, Supplementary Fig. 19 ) for the interaction of 2- α with CAN from UV–vis titration experiments, it is expected that 3- α would account for ~80% of the iron in the Raman samples. Therefore, the 822 cm −1 ν Fe=O vibration observed in the 9-CAN samples must arise mainly from 3- α . Notably, a second feature of similar intensity appears at 677 cm −1 with 413.1 nm excitation in the sample of 3- α ( Fig. 5b ). This lower-frequency feature persists when 3- α is probed with 514.5 nm excitation, a wavelength at which only 3- α has an absorption feature, but the 822 cm −1 vibration is not observed, consistent with the absorption features associated with the Fe IV =O unit [26] , [27] . With either excitation wavelength, the 677 cm −1 peak downshifts to 643 cm −1 on replacing H 2 16 O by H 2 18 O, but is not affected when the experiment was carried out in D 2 O ( Supplementary Figs 32–33 ). The 34 cm −1 downshift is consistent with a diatomic Fe–O vibration, but the lower frequency indicates a weaker Fe–O bond that is also resonance-enhanced with 514.5 nm excitation on Ce-adduct formation. Fe–O modes in this frequency range have previously been reported for complexes with Fe III (μ-O) 2 Fe IV (666 cm −1 ) [28] , [29] and Fe IV 2 (μ-O) 2 (674 cm −1 ) [30] cores, respectively, suggesting the possibility of forming an analogous Fe IV (μ-O) 2 Ce IV core, which would be consistent with the elemental composition of 3- α determined by CSI-HRMS. To test whether this feature could arise from an Fe IV (μ-O) 2 Ce IV diamond core, rR experiments on 3- α were performed in a 1:1 H 2 16 O:H 2 18 O solvent mixture. Under these conditions, the rR spectrum exclusively shows peaks at 677 and 643 cm −1 , with no peak found at an intermediate frequency that could be associated with a mixed-labelled diamond core (See Supplementary Fig. 32 ) [31] . The H 2 16 O:H 2 18 O experiment thus excludes formation of an Fe IV (μ-O) 2 Ce IV core. We have also considered the possibility that the 677 cm −1 vibration may correspond to the Fe–OH–Ce mode of an O=Fe IV –OH–Ce IV core, as earlier postulated [5] . However, two points argue against this possibility: (a) the lack of a D 2 O effect on the 677 cm −1 vibration [32] and (b) more importantly, the fact that Fe–OH–Fe vibrations are typically found in the range of 400–500 cm −1 (refs 32 , 33 ) much lower than observed for 3-α . Consideration of the above points together with its mass spectral formulation leads us to favour an O=Fe IV –O–Ce IV core for 3-α . An analogous heterodimetallic Fe IV –O–Sc III unit has been characterized crystallographically by Fukuzumi and Nam [34] , but unfortunately there is no Raman data reported for comparison. Identification of 3- α with an O=Fe IV –O–Ce IV core as the key reaction intermediate in WO reactions introduces unconsidered mechanistic scenarios for the oxidation of water by Ce IV ( Fig. 7 ). Most obviously, Ce IV appears not to behave simply as an outer-sphere oxidant, but instead forms an inner-sphere Fe IV (μ-O)Ce IV intermediate that is crucial for the reaction to proceed. Therefore, Ce IV -driven Fe-based WO activity not only requires the presence of two cis -labile sites but also a structure of the iron complex that allows formation of the Fe IV (μ-O)Ce IV intermediate. In this regard, the contrasting reactivities of 1- α and 1- β may arise from differences in their steric or electronic properties. A possible rationale comes from the differences in the nature of the donor trans to the cis -labile sites of the α and α isomers. While the α isomer has two tertiary amines trans to the labile positions, the β isomer has one tertiary amine and one pyridine. From our earlier survey of non-haem iron WO catalysts, the more active complexes are similar to 1- α with two tertiary amines trans to the two labile sites, whereas 1- β , like the [Fe II (CF 3 SO 3 ) 2 (tpa)] complex (tpa=tris(2-pyridylmethyl)amine), has lower WO activity [4] . In contrast, close inspection of the crystallographic data for 1- β (ref. 19 ) shows that the N-Me groups point towards the cis -labile sites in such a way that might inhibit for formation of oxo-bridged dinuclear species ( Supplementary Fig. 34 ). Although examination of simple β -[(mcp)Fe IV ( μ -O)Ce IV (NO 3 ) 3 ] + models seems to discard this possibility, a survey of the literature reveals that 1- α can form a number of oxo-bridged diferric complexes that have been crystallographically characterized, but dimeric species derived from 1- β are at present not known [35] . 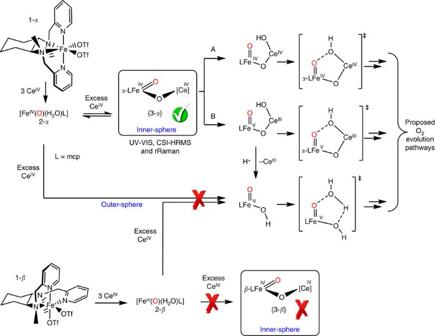Figure 7: Reactivity differences between topological isomers α-β. The mechanism is based on the formation of3-αas key intermediate for the O2evolution. Mechanismadescribes the oxo/oxyl radical coupling between FeIV(O) and CeIV(OH). Path (b) describes the formation of FeV(O) and the subsequent nucleophilic attack of a water molecule. Figure 7: Reactivity differences between topological isomers α-β. The mechanism is based on the formation of 3- α as key intermediate for the O 2 evolution. Mechanism a describes the oxo/oxyl radical coupling between Fe IV (O) and Ce IV (OH). Path ( b ) describes the formation of Fe V (O) and the subsequent nucleophilic attack of a water molecule. Full size image How intermediate 3- α evolves further to produce O 2 remains unclear [36] . In Fig. 7 are postulated two possible mechanism an oxo/oxyl radical coupling mechanism to form the O–O bond (Path a , Fig. 7 ) [12] and the alternative hypothesis entailing electron transfer from Fe IV to Ce IV to generate a highly electrophilic {Fe V (O)(μ-O)Ce III } oxidant ( Fig. 7 , path b ). Water binding to the Ce III would position it well for electrophilic attack by the Fe V =O moiety to form the O–O bond. This pathway is analogous to that proposed for 1 -catalysed C-H and C=C oxidations with Ce IV as an oxidant [37] . Also supporting the notion of a highly electrophilic oxidant are the observed effects of substituents on the pyridine of the supporting ligand of a related catalyst on WOC efficacy, where more electron withdrawing substituents on the pyridine ligand enhance both TON and TOF for water oxidation [5] . Nevertheless, at this point it is not possible to discard the other scenarios unequivocally. The [Fe IV (O)(μ-O)Ce IV ] intermediate we have characterized resembles the corresponding Mn V (O)( μ -O)Ca II (OH 2 ) unit proposed in some mechanistic models for the OEC ( Fig. 8 ), [38] , [39] , [40] making 3- α an iron-based functional OEC model. In fact, the resemblance becomes stronger with electron transfer from Fe IV to Ce IV to generate an [Fe V (O)(μ-O)Ce III ] oxidant. The strong similarities between iron and manganese chemistry in biologically relevant oxidation reactions suggest that this analogy should not be unexpected. Also relevant is the fact that Ce III can replace Ca II in biomolecules or act as an antagonist in pharmacology [41] , [42] , [43] . For example, it has been found that lanthanides, Ce in particular, are essential for the growth of Methylacidiphilum fumariolicum SoIV [41] , while Ca II can be replaced by Ce III in the pyrroloquinoline quinone (PQQ)-dependent methanol dehydrogenanse (MDH) enzymes to elicit superior catalytic properties [41] , [42] . 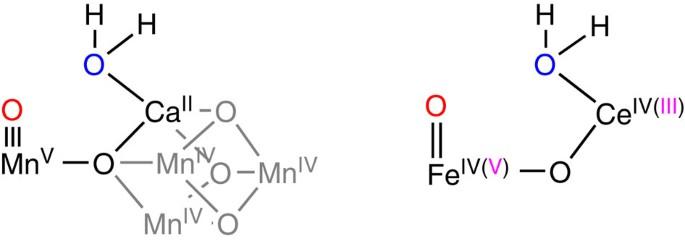Figure 8: Structure of the active species and analogy to the proposed intermediate of the OEC. Analogy between a proposed oxygen evolving complex intermediate and the iron-cerium adduct (3-α), both active species for the water oxidation, containing a metal in a high oxidation state and a Lewis acid, which may orientate the water molecule for the nucleophilic attack. Figure 8: Structure of the active species and analogy to the proposed intermediate of the OEC. Analogy between a proposed oxygen evolving complex intermediate and the iron-cerium adduct ( 3- α ), both active species for the water oxidation, containing a metal in a high oxidation state and a Lewis acid, which may orientate the water molecule for the nucleophilic attack. Full size image The mechanisms for O–O bond formation currently being considered for the OEC can be grouped in two main paths: (a) a nucleophilic attack of a water molecule to a Mn V ≡O (or a Mn IV -oxyl, Mn IV =O·) unit, and (b) an oxo/oxyl radical coupling mechanism [40] , [44] , [45] . Remarkable mechanistic insight into the O–O bond formation reaction has been obtained from studies of Mn (refs 38 , 39 , 46 ) and Co (refs 47 , 48 , 49 , 50 ) tetrametallic cubane model complexes. Up to now these cubane OEC models generally support the oxo/oxyl radical coupling mechanism to form the O–O bond. However, there are no catalytically active WO models that include in their structure a Lewis acid to mimic the role of Ca II in PSII (refs 38 , 39 , 46 , 51 , 52 ), despite the fact that a Lewis acid (Ca II , but also Sr II ) [53] , [54] has been proven to be absolutely required for the operation of the OEC. Given their obvious interest, the absence of heterodimetallic complexes that are active in water oxidation may reflect the extraordinary difficulty in accessing well-defined models where both a first row transition metal centre and a Lewis acid work together in water solution [50] . The success of our effort to trap and characterize 3- α as having an [O=Fe IV -O-Ce IV ] core that resembles the fundamental Mn V (O)( μ -O)Ca(OH 2 ) 2 structural motif of the OEC unit is therefore remarkable from an inorganic synthesis perspective. More importantly, the identification of an [O=Fe IV -O-Ce IV ] core that is active in water oxidation provides a model compound to study the formation of the O–O bond in detail. In conclusion, this work provides experimental evidence and characterization of an Fe IV –O–Ce IV species as the last detectable intermediate in Fe-catalysed WO reactions. Although Ru–O–Ce intermediates have been proposed in water oxidation reactions by different research groups [55] , [56] , [57] , [58] , to the best of our knowledge this is the first direct experimental characterization of a heterodimetallic core in a synthetic WO catalyst. Furthermore, the Fe IV –O–Ce IV active species we have described in this work can be construed as the closest structural and functional model for the essential heteodimetallic Mn V –O–Ca II centre involved in the water oxidation event in PSII. Materials Reagents were purchased from commercial sources and used as received, without any further purification. Cerium(IV) ammonium nitrate (CAN) (≥99.99%) and trifluoromethanesulfonic acid (ReagentPlus grade ≥99%) were purchased from Sigma-Aldrich. Solvents were purchased from SDS and Scharlab, purified and dried by passing through an activated alumina purification system (MBraun SPS-800) and stored in an anaerobic glovebox under N 2 . Complexes 1- α and 1- β were prepared as previously described. Water (18.2 MΩ cm) was purified with a Milli-Q Millipore Gradient AIS system. Physical methods UV–vis-NIR spectra were recorded on an Agilent 8453 diode array spectrophotometer (190–1,100 nm range) in 1-cm quartz cells. A cryostat from Unisoku Scientific Instruments was used for temperature control. The amount of gas generated was measured with a differential pressure transducer sensor (Honeywell-ASCX15DN, ±15 psi). Each reaction had its own reference reaction, which was connected to the other port of the sensor. Further details of the equipment are available elsewhere [4] , [5] . High resolution mass spectra High resolution mass spectra were recorded on a Bruker MicrOTOF-Q II instrument with ESI or Cryospray ionization sources at Serveis Tècnics of the University of Girona. Samples were introduced into the mass spectrometer ion source by direct infusion using a syringe pump and were externally calibrated using sodium formate. The instrument was operated in the positive ion mode. Resonance raman spectroscopy Resonance Raman (rR) spectra were collected via excitation with Kr + and Ar + lasers (Spectra-Physics BeamLok 2060-RM) and an Acton AM-506M3 monochromator equipped with a Princeton Instruments ACTON PyLON LN/CCD-1340 × 400 detector. Low-temperature spectra in H 2 O:CH 3 CN solution mixtures were obtained at 265 K using a 90° backscattering geometry. Raman frequencies were calibrated to indene before data collection. Rayleigh scattering was attenuated using a holographic notch filter (Kaiser Optical Systems) for each excitation wavelength. The monochromator slit width was set for a band pass of 4 cm –1 for all spectra. All spectra were collected using a laser excitation power of 100 mW. The plotted spectra are averages of 96 scans with collection times of 20 s. All spectra were intensity-corrected to the 922 cm –1 peak of the CH 3 CN solvent. Kinetic studies The required amount of iron complex was dissolved with 2.7 ml of Milli-Q water in a quartz UV–vis cell at 25 °C. Then, the Fe IV (O)(H 2 O) intermediate was generated by the addition of 3 equiv. of CAN dissolved in 50 μl of diluted HOTf (3:10, HOTf:H 2 O). Once fully formed, Milli-Q water (0.25 ml) was added to the solution. A second addition of CAN in 0.3 ml of HOTf:H 2 O (at pH~0) was added. This second addition leads to the desired final concentration of Ce IV (ranged from 1.25 to 18.75 mM) and iron complex (0.1 mM) for the kinetic studies at pH=1. Cerium(IV) consumption was monitored at λ =420 nm. Oxygen evolution was monitored in parallel by a pressure transducer. The initial rate method was applied to obtain rate constants in the kinetic studies to avoid interference of the consumption of the catalysts during the catalytic reactions. All the kinetic data were treated following the same procedure. Only data obtained within the first 10 s of reaction was used, which corresponds to the decay of 20% of the starting Ce absorbance. From these data, the self-decay of a Ce IV blank experiment (same concentration, pH=1) was subtracted. For the transformation of the absorbance to concentration, blank samples for every Ce IV concentration were linearized and the equation was used as a calibration curve. How to cite this article: Codolà, Z. et al . Evidence for an oxygen evolving iron–oxo–cerium intermediate in iron-catalysed water oxidation. Nat. Commun. 6:5865 doi: 10.1038/ncomms6865 (2015).